A synthetic nanomaterial for virus recognition produced by surface imprinting Major stumbling blocks in the production of fully synthetic materials designed to feature virus recognition properties are that the target is large and its self-assembled architecture is fragile. Here we describe a synthetic strategy to produce organic/inorganic nanoparticulate hybrids that recognize non-enveloped icosahedral viruses in water at concentrations down to the picomolar range. We demonstrate that these systems bind a virus that, in turn, acts as a template during the nanomaterial synthesis. These virus imprinted particles then display remarkable selectivity and affinity. The reported method, which is based on surface imprinting using silica nanoparticles that act as a carrier material and organosilanes serving as biomimetic building blocks, goes beyond simple shape imprinting. We demonstrate the formation of a chemical imprint, comparable to the formation of biosilica, due to the template effect of the virion surface on the synthesis of the recognition material. The design of artificial molecular recognition (nano)materials is an active field in the chemical sciences, with applications ranging from medical diagnostic [1] , [2] and environmental monitoring [3] to national security [4] . Since the advent of supramolecular chemistry in the 1980s, considerable effort has been invested in developing molecules that possess defined, predictable recognition properties [5] , [6] , [7] . Special focus has been placed on macrocyclic molecules, which have been shown to possess remarkable recognition properties with respect to anions [8] , cations [9] and small neutral molecules [10] . However, owing to a size discrepancy between host and guest molecules that is typically one to two orders of magnitude, applications with larger targets, such as proteins [2] , [11] , [12] , are limited. Molecular imprinting represents an alternative approach to the design of materials that possess specific molecular recognition properties [13] , [14] . It is based on the formation of a supramolecular complex of organic monomers together with a template molecule before polymerization. This procedure enables the three-dimensional positioning of the recognition units in the produced organic polymer [15] , [16] . Inorganic molecularly imprinted materials have also been developed. For instance, Katz and David [15] reported on the imprinting of bulk microporous silica. The originality of their approach lies on the choice of a building block that was used to occupy the micropores and to attach the functional groups to the walls of those pores. The so-produced materials were shown to possess shape-selective catalytic properties. In spite of promising prospects for molecular imprinting, applications involving voluminous biomolecular targets are hindered by the difficulty that arises when large biomolecules need access to binding sites within the produced polymer [17] . Nevertheless, examples of molecularly imprinted materials for biomolecular recognition have been developed for proteins [18] , [19] , [20] , [21] , [22] , [23] , [24] , [25] . The most convincing examples had been developed using surface-imprinting approaches. The imprinting of even bigger biomolecular entities, such as viruses, is of great interest, with possible applications in purification, diagnostics and therapy. Such imprinting also becomes more challenging as target size increases. Few examples of virus imprinting using organic polymers have been reported [26] , [27] , [28] , [29] , [30] . Nevertheless, the performances of the materials produced are still fairly limited and virus imprinting remains a great challenge when the intent of the design is ‘artificial antibodies’ that bind viral particles. Such synthetic systems would undeniably find a number of possible applications, from virus production and diagnostics to, ultimately, therapy. Herein, we report a synthetic strategy leading to an artificial organic–inorganic nanoparticulate material that possesses virus imprints on its surface and that we name virus-imprinted particles (VIPs). The method to produce VIPs is based on an sequential procedure consisting of three steps: (i) binding the template virus on the surface of a carrier material (here, silica nanoparticles, SNPs), (ii) incubating these virus-modified nanoparticles with a mixture of organosilanes, followed by the poly-condensation of the latter to grow an organosilica (silsesquioxane) recognition layer thereby forming a replica of the virus; and (iii) removing the template to free the imprints ( Fig. 1 ). The possibility of controlling the kinetics of layer growth is demonstrated to enable the control of the size of the imprints and, hence, the number of interaction points with the virion surface, ultimately permitting control of the affinity of the material for its template. 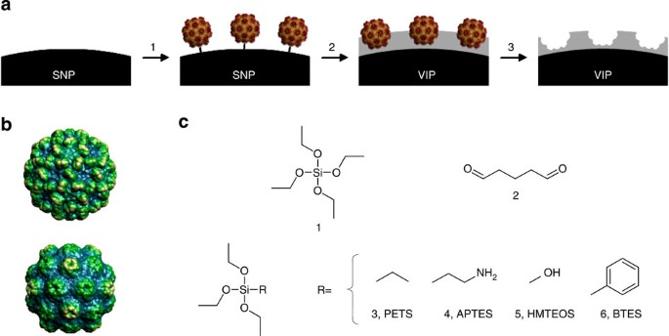Figure 1: Principle of preparation and materials used in the synthesis. (a) Step 1: immobilization of template virions at the surface of SNPs (in black); Step 2: addition of an OM to build the recognition layer (in grey); Step 3: removal of immobilized virions to free the virion imprints. (b) Images of the surface of the virions of TBSV (top) and TYMV (bottom) computed using VIPER particle ExploreR2(39). (c) Structures of 1: tetraethyl-orthosilicate, 2: glutaraldehyde, 3: PTES, 4: APTES, 5: HMTEOS and 6: BTES. Figure 1: Principle of preparation and materials used in the synthesis. ( a ) Step 1: immobilization of template virions at the surface of SNPs (in black); Step 2: addition of an OM to build the recognition layer (in grey); Step 3: removal of immobilized virions to free the virion imprints. ( b ) Images of the surface of the virions of TBSV (top) and TYMV (bottom) computed using VIPER particle ExploreR 2 ( [39] ). ( c ) Structures of 1: tetraethyl-orthosilicate, 2: glutaraldehyde, 3: PTES, 4: APTES, 5: HMTEOS and 6: BTES. Full size image VIPs synthesis and characterization As the carrier material to design the VIPs, we used highly monodisperse SNPs produced following the method developed by Stöber [31] . The statistical analysis of micrographs acquired using high-resolution field-emission scanning electron microscopy (FESEM) revealed a mean diameter of 410 nm. The high propensity of those nanoparticles to self-assemble into three-dimensional colloidal arrays represents an additional evidence of their high monodispersity ( Fig. 2a ). 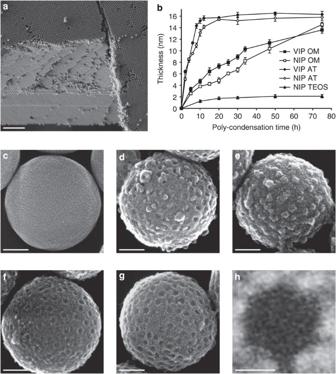Figure 2: Representative FESEM micrographs and layer growth kinetics. (a) Colloidal self-assembled three-dimensional arrays formed by the starting SNPs, (b) growth kinetics of the recognition layer as a function of the poly-condensation reaction time (mean±s.e.m.). Nanoparticles as they appear (c) before and (d,e) after growth of the recognition layer; (d) VIPsATand (e) VIPsOM, both with 8 nm-thick recognition layers. (f,g) Micrographs of VIPsOMand VIPsATonce the virions were removed; (h) Close-up view of a VIPsOM. Scale bars represent:a, 5 μm;c–g, 100 nm; andh, 10 nm. Figure 2: Representative FESEM micrographs and layer growth kinetics. ( a ) Colloidal self-assembled three-dimensional arrays formed by the starting SNPs, ( b ) growth kinetics of the recognition layer as a function of the poly-condensation reaction time (mean±s.e.m.). Nanoparticles as they appear ( c ) before and ( d , e ) after growth of the recognition layer; ( d ) VIPs AT and ( e ) VIPs OM , both with 8 nm-thick recognition layers. ( f , g ) Micrographs of VIPs OM and VIPs AT once the virions were removed; ( h ) Close-up view of a VIPs OM . Scale bars represent: a , 5 μm; c – g , 100 nm; and h , 10 nm. Full size image The first step in VIPs synthesis consisted of grafting the template virions on the surface of the SNPs. In order to provide anchoring amine moieties for this cross-linking, the SNPs were partially modified with aminopropyltriethoxysilane (APTES). A low density of amine groups at the SNP surface is essential to leave enough silanol groups for the further surface-initiated poly-condensation of the recognition layer. Further coupling of the virions was carried out in water using glutaraldehyde as a homo-bifunctional crosslinker. We used two small RNA plant viruses as model viruses. Tomato bushy stunt virus (TBSV) and turnip yellow mosaic virus (TYMV) are non-enveloped, icosahedral, single-stranded RNA viruses ( Fig. 1b ). Their capsids are made of 180 copies of protein subunits, with a mass of 40 kDa for TBSV and 20 kDa for TYMV [32] . The virions have diameters of 33 and 28 nm, molecular weights of 9.0 × 10 3 and 5.5 × 10 3 kDa, and isoelectric points of 4.1 and 3.8, respectively. Once the virions were bound, a silsesquioxane layer was grown from the surface of the SNPs. To produce this recognition layer by following a protein mimetic approach, we selected organosilanes that mimic the lateral chains of amino acids known to be of importance in protein–protein interactions ( Fig. 1c ) [33] , [34] . We hypothesized that these building blocks will self-assemble at the surface of the virions before their covalent incorporation within the recognition layer. This was expected to improve the recognition properties of the VIPs by creating not only a shape but also a chemical imprint that is complementary to the surface of the virion. Hereinafter, the term VIPs OM stands for particles imprinted with TYMV virions and having a recognition layer composed of an organosilanes mixture (OM), and the term non-imprinted particles (NIPs) OM for NIPs produced in the absence of template using the same OM. As controls, we selected two additional formulations, one with tetraethyl orthosilicate (TEOS) alone and one with a mixture of APTES and TEOS (AT). The corresponding VIPs are abbreviated VIPs AT for TYMV-imprinted particles having a recognition layer made of AT, and NIPs AT for those produced under the same conditions in the absence of template. The kinetics of surface-initiated growth of the silsesquioxane recognition layer in water at 10 °C followed by FESEM revealed that the thickness of the external layer reached only 2 nm after 75 h when the poly-condensation reaction was performed with TEOS alone ( Fig. 2b ). In the presence of APTES, the layer was 15 nm thick after 10 h. This faster growth can be safely attributed to the catalytic effect of the primary amine function of APTES on the hydrolysis of the organosilanes [35] . The size of the particles prepared with the mixture of organosilanes increased according to a sigmoidal function; the layer thickness reached 14 nm after 75 h ( Fig. 2b ). The slower kinetics as compared with that of the APTES/TEOS mixture may be explained by the lower amount of APTES present in a constant total amount of organosilanes. These results demonstrate the possibility of growing an organosilanes layer at the surface of the nanoparticles under aqueous conditions. They also confirmed that neither the crosslinking chemistry of the SNPs (using APTES and glutaraldehyde) nor the presence of the virions at the surface of the SNPs hampered this growth. An examination of the morphology of the particles produced with AT reveals the presence of open cavities with an average diameter of ~20 nm at the surface of the VIPs for a layer thickness of 8 nm ( Fig. 2d ). This suggests that the growth of the layer had started at the surface of the SNPs but was hindered by the virions, resulting in the formation of crater-like imprints ( Fig. 2d ). The virions were destroyed by the physical treatment of the particles before and/or during the FESEM imaging, thus leaving empty imprints. Particles synthesized in the presence of the silane mixture were distinguishable from predecessors by the presence of protuberances measuring about 32 nm in diameter ( Fig. 2e ) and by a thin shell around every virion that was not removed under FESEM sample preparation and imaging conditions. Thus, poly-condensation started not only at the surface of the SNPs but also at the surface of the virions that act as a template for this reaction. This observation supported our hypothesis that the selected silanes interacted with the entire surface of the virions before they were incorporated in the recognition layer. The ability of silicatein proteins to act as templates/catalysts for the biomineralization of silica has been demonstrated [36] . Numerous biomimetic synthetic silica systems have been reported and are mainly based on the modification of the protein to introduce catalytic/template sequences [36] , [37] , [38] . Here, we demonstrated that the template effect could be obtained by using a mixture of organosilanes that self-assemble around the native virus. By submitting these VIPs to an ultrasonic treatment under acidic conditions, this shell was broken without altering the recognition layer. FESEM micrographs showed that the protuberances observed previously were eliminated ( Fig. 2f ). The cleaned particles exhibited empty cavities at their surface, meaning that the virus imprinting method was successful. Also, the particles produced using the APTES/TEOS mixture resulted in being completely cleaned after the ultrasonic treatment ( Fig. 2g ). Images of the cavities taken at a higher magnification revealed their hexagonal shape (with an edge length of 11 nm), which originated from that of the template virus ( Fig. 2h ). Altogether, these results confirmed that the three-dimensional icosahedral architecture of the template virions was preserved under the mild conditions used throughout the full chemical synthesis. Virus-binding assays The binding performances of the synthesized VIPs were assessed in aqueous batch rebinding assays. VIPs and NIPs were incubated with TBSV or TYMV virions under well-defined conditions and, following centrifugation, the proportion of unbound virions was quantified using an enzyme-linked immunosorbent assay (ELISA) ( Fig. 3 ). 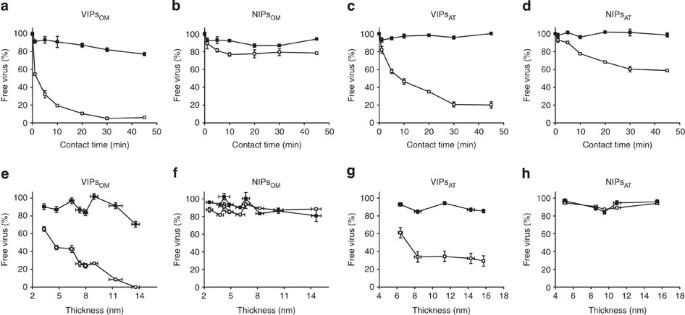Figure 3: Binding of virions of the templated TYMV and non-templated TBSV to VIPs and NIPs. Symbols are for TYMV (open squares) and for TBSV (solid squares). Binding time, selectivity, composition and thickness of the recognition layer were compared. (a–d) Four types of particles were assayed: (a) VIPsOM, (b) NIPsOM, (c) VIPsATand (d) NIPsAT; OM and AT particles with 8-mm-thick recognition layers. (e–h) Nanoparticles with recognition layers of increasing thicknesses (mean±s.e.m.) were assayed: (e) VIPsOM, (f) NIPsOM, (g) VIPsATand (h) NIPsAT. All values are presented normalized in percentage of initial virus concentration (mean±s.e.m.). Figure 3: Binding of virions of the templated TYMV and non-templated TBSV to VIPs and NIPs. Symbols are for TYMV (open squares) and for TBSV (solid squares). Binding time, selectivity, composition and thickness of the recognition layer were compared. ( a – d ) Four types of particles were assayed: ( a ) VIPs OM , ( b ) NIPs OM , ( c ) VIPs AT and ( d ) NIPs AT ; OM and AT particles with 8-mm-thick recognition layers. ( e – h ) Nanoparticles with recognition layers of increasing thicknesses (mean±s.e.m.) were assayed: ( e ) VIPs OM , ( f ) NIPs OM , ( g ) VIPs AT and ( h ) NIPs AT . All values are presented normalized in percentage of initial virus concentration (mean±s.e.m.). Full size image The results of the binding experiments revealed that, starting from an initial virus concentration of 65 pM, after 30 min, as much as 95% of TYMV were bound to VIPs OM possessing 8-nm-thick recognition layers (834 μg ml −1 or 100 μg per 120 μl; Fig. 3a ). Under the same conditions, these nanoparticles after 30 min bound no more than 12% of TBSV ( Fig. 3a ). Thus, VIPs OM specifically bind the template virions and almost none of the virions of another icosahedral virus possessing a comparable particle diameter and isoelectric point. Quantification of the intrinsic binding of NIPs possessing the same chemical composition as VIPs but having no imprints resulted in 21% of TYMV virions and 6% of TBSV virions bound after 45 min, respectively ( Fig. 3b ). Thus, TYMV adsorbs on NIPs OM more than TBSV does, but the difference between both viruses is too small to explain the strong effect observed with the VIPs OM . The selectivity of the VIPs, at a target concentration in the pM range, is essentially owing to the presence of the virion imprints at the surface of the nanoparticles. To assess the influence of the chemical composition of the recognition layer, VIPs with an 8 nm recognition layer synthesized with AT were assayed under the same conditions. VIPs AT bound 80% of the TYMV virions in 30 min while binding of TBSV virions was <5% ( Fig. 3c ). As for NIPs, they bound significantly more TYMV virions (that is, 40% in 30 min) than TBSV virions (5% in 30 min), showing that their binding performances were lower than those of the VIPs prepared with an APTES/TEOS mixture ( Fig. 3d ). This pointed to the importance of the chemical composition of the recognition layer and supported our hypothesis of an organosilanes chemical imprinting. According to our initial hypothesis, increasing the recognition layer thickness (limited to the radius of the virion) should significantly increase the surface area available for interactions per virion and, hence, the number of potential interaction points between hosts and guests. To verify the influence of the thickness of the recognition layer on the affinity of VIPs for their template, we produced VIPs OM and VIPs AT with layers of various thicknesses. In batch assays, the binding of the template to the VIPs OM increased with the thickness of the recognition layer (625 μg ml −1 or 75 μg per 120 μl). The fraction of bound virus reached 34% for a layer thickness of 3 nm, 74% for one of 9 nm and 100% for a layer of 14 nm ( Fig. 3e ). The non-template virus (TBSV) was bound only to a limited extent to particles with thin recognition layers: 10% of the non-template virus, while particles with a layer of 14 nm had bound to 30%. In binding assays done with NIPs OM ( Fig. 3f ), only about 10% of each virus was bound. VIPs AT particles bound specifically to their template ( Fig. 3g ), and there was no major effect from recognition layer thickness. As much as 40% of the virions of TYMV were bound to particles with a recognition layer of 6 nm and 70% to the particles with recognition layers of 8, 11, 14 or 16 nm. None of the NIPs AT bound either virus ( Fig. 3h ). Again, these results confirmed that the affinity of the VIPs material for its template virus can be tuned by varying the thickness of the recognition layer. Competition binding assay in serum and rebinding To assess the selectivity of the VIPs OM and the effect of a more complex matrix, we performed competition binding assays in buffer and human serum (HS) at different dilutions ( Fig. 4a ). HS is a complex matrix possessing, in addition to a high total protein concentration (60–85 g l −1 , predominantly albumin and immunoglobulins), lipids, metabolites, vitamins, regulatory factors and electrolytes. It has to be added that for non-diluted HS, the ELISA test used did not show a consistent response and therefore prevented us from evaluating the VIPs OM -binding performances in these conditions. The assays performed in buffer revealed that 84% of the template TYMV was bound to VIPs OM while only 10% of the non-template TBSV was bound to the particles. This result confirmed the selectivity of VIPs OM for its template. The competition assays performed in HS showed that VIPs OM are specifically binding 45, 64 and 88% of the template TYMV at 1:10, 1:50 and 1:100 HS dilutions, respectively. The non-template TBSV binding on the particles is of 6, 16 and 18% at 1:10, 1:50 and 1:100 HS dilution, respectively. These results confirmed that the VIPs OM maintained their capabilities of discriminating between the two viruses in complex matrix, such as HS. 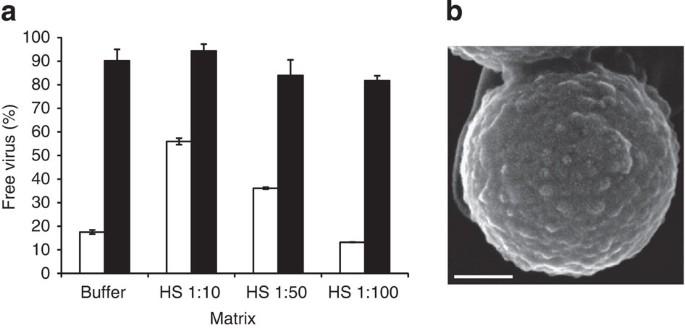Figure 4: Competition binding assay of the templated TYMV and non-templated TBSV to VIPsOMin complex matrices and FESEM of VIPsOMafter a rebinding assay. (a) Symbols are for TYMV (white bars) and for TBSV (black bars). The competition assays were performed with VIPsOMparticles with a 8-nm-thick recognition layer in buffer containing bovine serum albumin (75 μg ml−1) and in different dilution of HS (1:10, 1:50 and 1:100). All values are presented normalized in percentage of initial virus concentration (mean±s.e.m.). (b) VIPsOMparticles after the binding assay with the template TYMV. Scale bar represent 100 nm. Figure 4: Competition binding assay of the templated TYMV and non-templated TBSV to VIPs OM in complex matrices and FESEM of VIPs OM after a rebinding assay. ( a ) Symbols are for TYMV (white bars) and for TBSV (black bars). The competition assays were performed with VIPs OM particles with a 8-nm-thick recognition layer in buffer containing bovine serum albumin (75 μg ml −1 ) and in different dilution of HS (1:10, 1:50 and 1:100). All values are presented normalized in percentage of initial virus concentration (mean±s.e.m.). ( b ) VIPs OM particles after the binding assay with the template TYMV. Scale bar represent 100 nm. Full size image In order to visualize the template rebinding on the VIPs OM , we collected a sample after the binding assay and processed it for FESEM acquisition ( Fig. 4b ). The micrograph suggested that the virions are occupying, as postulated, the imprints. In addition, the number of imprints is consistent with the number of protuberances observed on the particles surfaces after the binding assay. We developed a strategy to produce VIPs, a nanomaterial that possesses selective molecular recognition properties in the pM range for a non-enveloped icosahedral plant virus. This method relies on the fact that a silsesquioxane layer can be grown at the surface of SNPs in a manner that allows control of thickness and composition. We have demonstrated that the elements of recognition for the nanomaterial can be built using a mixture of organosilanes that mimic a series of natural amino acids, and that this allows the formation of not only geometrical but also chemical imprints of the virus. Evidence of this phenomenon was provided by comparative electron microscopy analyses of the produced particles and virus-binding experiments. In addition, we showed that the thickness of the recognition layer influences the affinity of the resulting material for its template, providing an additional parameter for tuning the properties of the VIPs. The binding performances in a more complex matrix (HS), in a virus competition configuration, confirmed the selectivity of the VIPs OM . We expect that the reported method can be applied to all icosahedral viruses; it represents a milestone in the production of purely synthetic materials that simultaneously possess high affinity and high selectivity for those viruses. Materials Tetraethyl orthosilicate (TEOS, ≥99%), (3-aminopropyl)-triethoxysilane (APTES, ≥98%), ammonium hydroxide (ACS reagent, 28–30%), ethanol (ACS reagent, anhydrous) and glutaraldehyde (Grade I, 25% in water) were purchased from Sigma-Aldrich (Switzerland). Hydroxymethyltriethoxysilane (HMTEOS, 50% in ethanol), n-propyltriethoxysilane (PTES, 97%) and benzyltriethoxysilane (BTES, 97%) were purchased from ABCR (Germany). All chemicals were used without further purification. Nanopure water (resistivity ≥18 MΩ cm) was produced with a Millipore Synergy purification system. TBSV and TYMVwere propagated and purified as described previously [32] . Filtered-sterilized human serum was purchased from Sigma-Aldrich. ELISA (double antibody sandwich) kits specific for TBSV or TYMV were purchased from AC Diagnostics (USA). SNPs synthesis The SNPs were prepared by adapting the procedure described elsewhere [20] as follows. All chemicals and solvents were equilibrated at 20 °C for 1 h in a water bath before use. Forty millilitres of ammonium hydroxide (28–30%) and 345 ml of ethanol were mixed in a 1 l round bottom flask, under stirring condition (600 r.p.m.). Fifteen millilitres of TEOS were added and the solution kept under stirring for 20 h. The resulting milky suspension was centrifuged at 3,220 g for 10 min and the white pellet resuspended in ethanol. This operation (hereafter called ‘washing cycle’) was repeated once with ethanol and thrice with water to yield 4 g of SNPs that were stored at 4 °C. VIPs synthesis In a typical synthesis experiment, 18 ml of 3.2 mg ml −1 of SNPs in water were reacted with 11 μl (0.047 mmol) of APTES for 30 min, in 20 ml glass vials under stirring condition (400 r.p.m.) in a water bath at 20 °C. After two washing cycles with nanopure water, the particles were incubated during 30 min in 18 ml of 1% (v/v) aqueous glutaraldehyde solution. After two washing cycles with nanopure water, they were then incubated with the template virus (at 0.05 mg ml −1 ) for 1 h under magnetic stirring. Subsequently, 18 μl (0.081 mmol), 36 μl (0.161 mmol) or 54 μl (0.242 mmol) of TEOS were added to the reaction mixture and allowed to react for 2 h to produce VIPs OM , VIPs AT or VIPs T , respectively. Temperature was then lowered at 10 °C and the relevant organosilane mixtures added. Samples were collected at increasing reaction times and purified as described in the Method section. To prepare particles with the OM, the following organosilanes were added sequentially to the reaction mixture: 9 μl (0.035 mmol) of BTES, 9 μl (0.039 mmol) of PTES, 18 μl (0.04 mmol) of HMTEOS and 9 μl (0.038 mmol) of APTES. Eighteen microlitres (0.077 mmol) of APTES were added to prepare particles with AT. During the preparation of particles with TEOS (T; NIPs only), no additional silane was added at this step. For the three different types of particles, samples were collected at increasing reaction times and washed twice with nanopure water and stored at 4 °C. All washing steps were performed by centrifugation at 3,220 g for 5 min and the pellets were resuspended by ultrasonic treatment for 2 min using an Elmasonic S30H ultrasonic bath. NIPs were produced in a similar fashion by omitting the virus addition step. Virus removal VIPs were suspended in the removal solution (1 M HCl and 0.01% v/v Triton-X 100) and subjected to an ultrasonic treatment as above but for 10 min at 30 °C. Under stirring conditions (600 r.p.m. ), the VIPs suspensions were incubated for 30 min at 40 °C. Subsequently, the so-treated VIPs were submitted to an additional ultrasonic treatment for 30 min, washed trice in nanopure water, centrifuged at 3,220 g for 5 min, freeze-dried and weighted using an ultra-microbalance (Mettler Toledo XP2U). Scanning electron microscopy and particle size measurement Particles were imaged using a Zeiss SUPRA 40VP scanning electron microscope. For neat VIPs and NIPs analyses, 2 μl of each sample were spread on freshly cleaved mica sheets, dried at ambient conditions and sputter-coated with a gold–platinum alloy for 15 s at 10 mA (SC7620 Sputter coater). For the VIPs OM after template (TYMV) binding, the particles were incubated with TYMV in the same conditions as for the virus-binding assay (see hereafter) and collected after 30 min contact time. Two microlitres of this suspension was spread on a freshly cleaved mica slide and sputter-coated as described above. Micrographs were acquired using the InLens mode with an accelerating voltage of 20 kV. Particle sizes were measured on micrographs acquired at a magnification of X150,000 using the Olympus Analysis software package. About 100 measurements were made per type of particles. Virus-binding assay In a typical experiment, a solution containing a virus at a concentration of 65 pM (for both single and competition binding assay), 10 mM sodium phosphate, 50 mM NaCl and 75 μg ml −1 of bovine serum albumin (final pH 5.8) was mixed with the particles at a concentration of 834 μg ml −1 unless otherwise mentioned in a final volume of 120 μl. The reaction medium was then incubated at 25 °C and shaken at 650 r.p.m. After the desired contact time, the suspension was centrifuged at 16,100 g for 1 min and 70 μl of the supernatant was withdrawn for virus quantification by a double antibodies sandwich ELISA assay performed following the manufacturer’s protocol. The measured values were compared with a standard curve obtained with solutions containing defined amounts of virus dissolved in the same buffer that for the interaction assay. For the competition assay performed in HS, solutions containing both template and non-template viruses at a concentration of 65 pM, 10 mM sodium phosphate, 50 mM NaCl and different dilutions of humans serum (1:10, 1:50 and 1:100) were mixed with the particles at a concentration of 834 μg ml −1 in a final volume of 120 μl. The resulting suspensions were incubated for 30 min at 25 °C, treated and analysed as for the binding assays performed in buffer (see above). The obtained values were compared with standard curves obtained with a mixture of both virus solutions containing defined amounts of virus in the same conditions (HS dilutions) that for the interaction assay. How to cite this article: Cumbo, A. et al . A synthetic nanomaterial for virus recognition produced by surface imprinting. Nat. Commun. 4:1503 doi: 10.1038/ncomms2529 (2013).